A light-driven sodium ion pump in marine bacteria Light-driven proton-pumping rhodopsins are widely distributed in many microorganisms. They convert sunlight energy into proton gradients that serve as energy source of the cell. Here we report a new functional class of a microbial rhodopsin, a light-driven sodium ion pump. We discover that the marine flavobacterium Krokinobacter eikastus possesses two rhodopsins, the first, KR1, being a prototypical proton pump, while the second, KR2, pumps sodium ions outward. Rhodopsin KR2 can also pump lithium ions, but converts to a proton pump when presented with potassium chloride or salts of larger cations. These data indicate that KR2 is a compatible sodium ion–proton pump, and spectroscopic analysis showed it binds sodium ions in its extracellular domain. These findings suggest that light-driven sodium pumps may be as important in situ as their proton-pumping counterparts. Microorganisms utilize ion-transporting microbial rhodopsins for light-energy conversion and light-signal transduction [1] , [2] . Light-driven outward proton and inward chloride pumps are used to create membrane potential for ATP synthesis [3] , [4] , [5] , while a light-gated ion channel depolarizes cells for phototaxis of Chlamydomonas [6] , [7] , [8] . These rhodopsins are important tools for optogenetics, where channelrhodopsin (ChR) excites neurons by light, and ion pumps are used for neural silencing [9] , [10] , [11] . The light-driven proton pump bacteriorhodopsin (BR) and chloride pump halorhodopsin (HR) were first discovered in 1971 (ref. 12 ) and 1977 (ref. 13 ), respectively, from Halophilic archaea. Since 2000, metagenomic analysis revealed that microbial rhodopsins are widely distributed among marine prokaryotes, most of which were classified as light-driven proton pumps (proteorhodopsin; PR) [2] , [14] , [15] , [16] . Although there were no data on the proton pump activity of PR in native marine bacteria, light-induced pH drops of native cell suspensions have been successfully recorded for flavobacteria [17] and γ-proteobacteria [18] . These facts suggest that the contribution of PR phototrophy is significant in marine environment, where light-driven proton pumps convert the energy of sunlight to proton gradients as the energy source of the cell. Similarly, sodium ion gradients are also widely used to drive uptake of nutrients [19] , [20] , but there have been no reports of a light-driven sodium ion pump. Possibility of HR as the outward sodium ion pump was originally discussed [13] , but it is now established that HR is an inward chloride pump [21] . Absence of sodium ion-pumping rhodopsins may be reasonable from the chemical point of view. All microbial rhodopsins possess an all- trans retinal as the chromophore, which binds to a lysine residue through a protonated retinal Schiff base (RSB) linkage ( Supplementary Fig. S1 ) [3] , [4] , [22] . Therefore, light energy is captured by the positively charged retinal chromophore. In case of BR and PR, transient drop of the RSB pKa by retinal photoisomerization causes the proton transfer to the extracellular side, and reprotonation from the cytoplasmic side leads to the outward proton pump [3] , [4] , [22] . In case of HR, chloride binding stabilizes the protonated RSB, and retinal photoisomerization alters the interaction of the ion pair, leading to the inward chloride pump [23] , [24] . In contrast, cations other than proton are probably unstable near the protonated RSB because of an electrostatic repulsion. Despite the above explanation has been generally accepted, we report the discovery of a light-driven sodium ion pump in this paper. The marine flavobacterium K. eikastus possesses two rhodopsins (KR1 and 2). While KR1 is a typical proton pump, KR2 pumps sodium ion outward. The sodium ion-pumping rhodopsin (NaR) can also pump lithium ion, but it becomes a proton pump in potassium chloride or salts of larger cations. KR2, a compatible sodium ion–proton pump, was converted to uni-functional sodium ion and proton pumps by mutations, from which important amino acids were revealed for sodium ion and proton pumps. The molecular mechanism of the light-driven sodium ion pump will be discussed. K. eikastus KR2 is a light-driven sodium ion pump We first measured light-driven pump activity in native cell suspensions of K. eikastus [25] , a marine Flavobacterium. The pump activity was monitored by a pH electrode at various growth phases. Although no pumping activity was observed before stationary phase (10 h in Fig. 1a ), the cells showed pH drop upon illumination at 96 h, which was abolished by the protonophore carbonylcyanide-m-chlorophenylhydrazone (CCCP). This reproduced our previous observation [17] , implying that K. eikastus contains a PR-like outward proton pump. However, at 48 h, we observed light-induced pH increase, which was not affected by CCCP ( Fig. 1a ). This result (pumping activities at all growth phases; Supplementary Fig. S2 ) suggests that there are multiple ion-pumping rhodopsins that function at different stages of the growth of K. eikastus . Genomic analysis shows two microbial rhodopsins in K. eikastus (KR1 and KR2), where KR1 belongs to PR-clade, and KR2 is located in an isolated clade of unknown function ( Fig. 1b and Supplementary Fig. S3 ; detailed phylogenic tree). It is suggested that KR1 and KR2 are the major gene products at 96 and 48 h, respectively, in Fig. 1a . 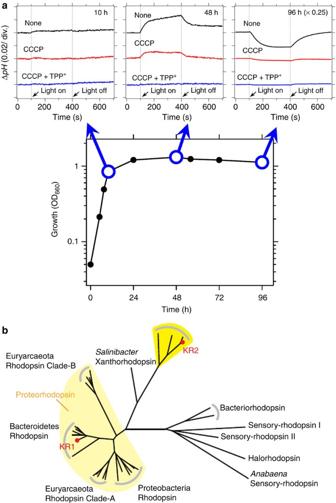Figure 1: Light-driven pump activity ofKrokinobacter eikastus. (a) Light-induced pump activity in nativeK. eikastuscell suspensions containing 100 mM NaCl is measured using a pH electrode (top; black lines). Cells are collected at 10, 48 and 96 h in the growth phase (bottom). Red and blue lines show the pump activities measured after the addition of CCCP and CCCP+TPP+, respectively. (b) Phylogenetic tree of microbial rhodopsins’ amino-acid sequences. KR1 and KR2 are indicated by red circles. Figure 1: Light-driven pump activity of Krokinobacter eikastus . ( a ) Light-induced pump activity in native K. eikastus cell suspensions containing 100 mM NaCl is measured using a pH electrode (top; black lines). Cells are collected at 10, 48 and 96 h in the growth phase (bottom). Red and blue lines show the pump activities measured after the addition of CCCP and CCCP+TPP + , respectively. ( b ) Phylogenetic tree of microbial rhodopsins’ amino-acid sequences. KR1 and KR2 are indicated by red circles. Full size image To study the function of the rhodopsins, C-terminal his-tagged KR1 or KR2 were overexpressed in Escherichia coli (C41 (DE3) strain). KR1 and KR2 show very similar absorption spectra ( Fig. 2a ), and the retinal configurations of both proteins are >90% all- trans form in both dark and light conditions ( Supplementary Fig. S4 ). Therefore, the all- trans isomer is the functional form as in the other microbial rhodopsins [1] . We then measured light-induced pH changes of E. coli cell suspensions containing KR1 or KR2. In case of KR1, we observed pH drop upon illumination, which was prevented by the protonophore CCCP ( Fig. 2b ). This indicates that KR1 is a light-driven proton pump, which is consistent with the phylogenic analysis ( Fig. 1b ). In contrast, we observed light-induced pH increase for KR2, which is accelerated with CCCP, but completely abolished with CCCP and tetraphenylphosphonium bromide (TPP + ) ( Fig. 2c ). This indicates that the protons move passively in response to a transmembrane electrical potential, and thus KR2 pumps an ion other than proton. Because of similar pH changes in E. coli cell suspensions ( Fig. 2b ), it is concluded that KR2 and KR1 are major products at 48 and 96 h, respectively, in the growth of K. eikastus ( Fig. 1a ). 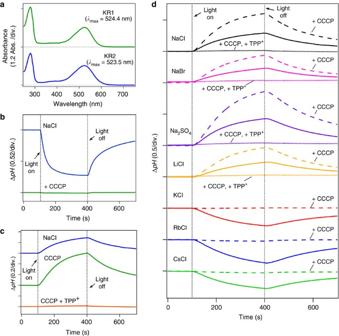Figure 2: Light-driven proton and sodium ion transport by KR1 and KR2. (a) Absorption spectra of purified KR1 and KR2 solubilized in the detergent DDM. (b) Pump activity ofE. colicell suspensions in 100 mM NaCl expressing KR1 without (blue) and with (green) CCCP. (c) Pump activity ofE. colicell suspensions in 100 mM NaCl expressing KR2. The activities after additions of CCCP (green) and CCCP+TPP+(orange) are shown. (d) Light-induced pump activity ofE. colicell suspensions (100 mM) of different salt solutions expressing KR2. The activities after additions of CCCP (dashed lines) and CCCP+TPP+(dotted lines) are shown. Figure 2: Light-driven proton and sodium ion transport by KR1 and KR2. ( a ) Absorption spectra of purified KR1 and KR2 solubilized in the detergent DDM. ( b ) Pump activity of E. coli cell suspensions in 100 mM NaCl expressing KR1 without (blue) and with (green) CCCP. ( c ) Pump activity of E. coli cell suspensions in 100 mM NaCl expressing KR2. The activities after additions of CCCP (green) and CCCP+TPP + (orange) are shown. ( d ) Light-induced pump activity of E. coli cell suspensions (100 mM) of different salt solutions expressing KR2. The activities after additions of CCCP (dashed lines) and CCCP+TPP + (dotted lines) are shown. Full size image KR2 pumps an ion other than proton similarly to HR, an inward chloride pump, for which identical light-induced pH changes were reported [21] . If KR2 is a chloride pumping rhodopsin, the pump activity must strongly depend on anions. However, light-induced pH changes were identical for the solution containing NaCl, NaBr and Na 2 SO 4 ( Fig. 2d ). It should be particularly noted that similar signal was obtained in Na 2 SO 4 , and HR does not pump SO 4 2− . In contrast to the observed anion independence, strong cation dependence was observed for KR2. Although the pump activity was similar in LiCl, light-induced pH drop was observed in KCl, RbCl and CsCl, which is prevented with CCCP ( Fig. 2d ). These results show that KR2 is an outward pump of sodium ion and lithium ion, but pumps proton in salts of K + , Rb + and Cs + . Under physiological conditions in the ocean, KR2 probably functions as light-driven NaR. Linear dependence of pumping activities on light power indicates that both sodium ion and proton pumps by KR2 are accomplished by a single-photon event ( Supplementary Fig. S5 ). The proton pump efficiency (16 proton KR2 −1 min −1 ) estimated from the initial slope of the pH change is much lower than that of BR (204 proton BR −1 min −1 ) and flavobacterial PR (124 proton PR −1 min −1 ) [17] , [26] . The proton-pumping microbial rhodopsins such as BR and PR have proton acceptor and donor to the protonated RSB in the C-helix, and the negatively charged proton acceptor also functions as the RSB counterion. They are D85 and D96 in BR [27] , [28] , and D97 and E108 in PR [29] , respectively. These carboxylic residues are replaced by neutral amino acids (N112 and Q123) in KR2, but the corresponding position of T89 in BR is D116 in KR2 ( Table 1 ). It seems that the RSB counterion is shifted one helix turn towards the cytoplasmic side in NaR ( Supplementary Fig. S6 ; complete sequences). While conventional proton pumps possess the DTD(E) motif, NaR has the NDQ motif. Table 1 Amino-acid sequences of the C-helix in various microbial rhodopsins (from R82 to D96 in BR numbering). Full size table K. eikastus KR2 binds sodium ions As KR2 is a light-driven sodium ion pump, NaR probably possesses a sodium-ion binding site. Chloride binds to HR as the RSB counterion, so that the binding can be monitored by colour change ( λ max change by >20 nm) [30] . In contrast, NaR shows little colour change between the presence and absence of sodium ions ( Fig. 3a and Supplementary Fig. S7 ), suggesting that the binding site is distant from the retinal chromophore. Absorption spectra are red shifted at low pH, presumably because of the protonation of the counterion (D116), while the complex titration curves suggest multiple pKa values in KR2 ( Supplementary Fig. S8 ). 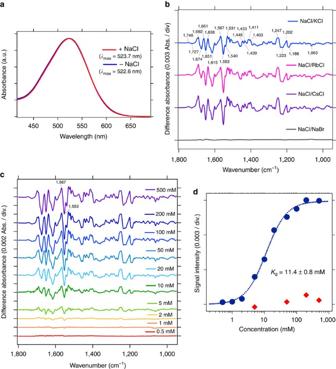Figure 3: Sodium ion binding to KR2. (a) Absorption spectra of KR2 in the presence (red) and absence (blue) of 100 mM NaCl. (b) ATF-FTIR difference spectra upon exchange of 50 mM NaCl/KCl (blue), NaCl/RbCl (pink), NaCl/CsCl (purple) and NaCl/NaBr (grey). (c) ATF-FTIR difference spectra for different concentrations of NaCl/KCl. (d) Salt concentration dependence for the peak height at 1553 and 1567, cm−1incat pH 8.0 (blue circles) and pH 3.6 (red diamonds). Figure 3: Sodium ion binding to KR2. ( a ) Absorption spectra of KR2 in the presence (red) and absence (blue) of 100 mM NaCl. ( b ) ATF-FTIR difference spectra upon exchange of 50 mM NaCl/KCl (blue), NaCl/RbCl (pink), NaCl/CsCl (purple) and NaCl/NaBr (grey). ( c ) ATF-FTIR difference spectra for different concentrations of NaCl/KCl. ( d ) Salt concentration dependence for the peak height at 1553 and 1567, cm −1 in c at pH 8.0 (blue circles) and pH 3.6 (red diamonds). Full size image We next studied sodium ion binding using attenuated total reflection-Fourier transform infrared (ATR-FTIR) spectroscopy at pH 8.0, which monitors infrared spectral changes upon cation exchange [31] . The difference spectrum between NaCl and NaBr coincides to the baseline ( Fig. 3b ), indicating no anion binding to KR2. In contrast, clear difference spectra were obtained between NaCl and KCl, which originates from cation binding. It should be noted that the exchanges of Na + to K + , Rb + or Cs + yielded identical spectra ( Fig. 3b ). As vibrational signals are highly sensitive to the environment [32] , this result suggests that none of K + , Rb + and Cs + binds to NaR. The difference spectra change in amplitude without shape change at different salt concentrations ( Fig. 3c ), which therefore monitors sodium ion binding, and we determined the dissociation constant ( K d ) to be 11.4 mM ( Fig. 3d ). Unlike neutral pH, no binding was observed at pH 3.6 ( Fig. 3d ), suggesting that protonation prevents binding of Na + . Photocycles during sodium ion and proton pumps in KR2 We next studied the photocycles during sodium ion and proton pumpings, where the KR2 protein is reconstituted into lipid bilayer ( Fig. 4 ) and solubilized in detergent ( Supplementary Fig. S9 ). In NaCl (Na + pump), red-shifted K, blue-shifted L M and red-shifted O intermediates appeared sequentially in the photocycle ( Fig. 4a–d and Supplementary Fig. S10 ; procedure of the reconstruction of the intermediate spectra). The present analysis shows that the L-like (505 nm) and M-like (400 nm) states appear simultaneously, unlike BR [33] and PR [34] . Since the rise of the O intermediate was accelerated at high NaCl concentrations ( Supplementary Fig. S11 ), uptake of the sodium ion probably occurs upon formation of the O intermediate ( Fig. 4d ). The photocycle of KR2 with lithium ion showed large O accumulation similar to sodium ion ( Supplementary Fig. S12 ). It should be noted that the retinal chromophore is positively charged, which provides high energy barrier for the sodium ion uptake. It is thereby likely that transient RSB deprotonation (M formation) assists the uptake. 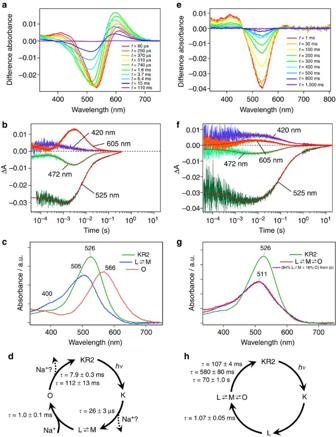Figure 4: Photocycles of KR2 for sodium ion pump activity. (a) Transient absorption spectra of KR2 reconstituted in DOPC in 100 mM NaCl at pH 8.0. (b) Time traces of absorption changes of KR2 in NaCl at 420 (blue), 472 (light green), 525 (green) and 605 nm (orange) probe wavelengths. Red lines indicate fitting lines based on the sequential kinetic model shown ind. (c) Absorption spectra of photointermediates in NaCl, which are calculated from decay-associated spectra. (d) Photocycle scheme of KR2 in NaCl determined by flash photolysis. Sodium ion uptake occurs upon formation of the O intermediate, while sodium ion release is expected to occur upon decay of the K intermediate or decay of the O intermediate (dashed arrows). The O decay is described by two time constants (τ1/e) of 7.9 ms (90.6%) and 112 ms (9.4%). (e) Transient absorption spectra of KR2 reconstituted in DOPC in 100 mM KCl at pH 8.0. (f) Time traces of absorption changes of KR2 in KCl at 420 (blue), 472 (light green), 525 (green) and 605 nm (orange) probe wavelengths. Red lines indicate the fitting lines based on the sequential kinetic model shown inh. (g) Absorption spectra of photointermediates in KCl calculated from decay-associated spectra. (h) Photocycle scheme of KR2 in KCl determined by flash photolysis. The time constant of the K decay is not determined as the decay signal is noisy. The recovery of KR2 is described by three time constants (τ1/e) of 107 ms (67.1%), 580 ms (24.2%) and 7.0 s (8.7%). Figure 4: Photocycles of KR2 for sodium ion pump activity. ( a ) Transient absorption spectra of KR2 reconstituted in DOPC in 100 mM NaCl at pH 8.0. ( b ) Time traces of absorption changes of KR2 in NaCl at 420 (blue), 472 (light green), 525 (green) and 605 nm (orange) probe wavelengths. Red lines indicate fitting lines based on the sequential kinetic model shown in d . ( c ) Absorption spectra of photointermediates in NaCl, which are calculated from decay-associated spectra. ( d ) Photocycle scheme of KR2 in NaCl determined by flash photolysis. Sodium ion uptake occurs upon formation of the O intermediate, while sodium ion release is expected to occur upon decay of the K intermediate or decay of the O intermediate (dashed arrows). The O decay is described by two time constants ( τ 1/ e ) of 7.9 ms (90.6%) and 112 ms (9.4%). ( e ) Transient absorption spectra of KR2 reconstituted in DOPC in 100 mM KCl at pH 8.0. ( f ) Time traces of absorption changes of KR2 in KCl at 420 (blue), 472 (light green), 525 (green) and 605 nm (orange) probe wavelengths. Red lines indicate the fitting lines based on the sequential kinetic model shown in h . ( g ) Absorption spectra of photointermediates in KCl calculated from decay-associated spectra. ( h ) Photocycle scheme of KR2 in KCl determined by flash photolysis. The time constant of the K decay is not determined as the decay signal is noisy. The recovery of KR2 is described by three time constants ( τ 1/ e ) of 107 ms (67.1%), 580 ms (24.2%) and 7.0 s (8.7%). Full size image In KCl (proton pump), the photocycle became >10 times slower and the accumulation of O was significantly decreased ( Fig. 4e–h ). KR2 does not possess a proton donor to RSB as D96N functions in BR [27] , which reasonably explains the long-lived proton pump cycle. However, in the case of D96 BR, the accumulation of O is negligible [27] . The measurable accumulation of O in the proton-pumping photocycle may suggest the 13- cis form as the chromophore structure of O in KR2. Mutational analysis of K. eikastus KR2 Finally, we replaced several amino acids to identify important residues for transport. We examined (i) the amino acids (R109, N112, D116, Q123 and D251) homologous to those involved in proton transport in BR (R82, D85, T89, D96 and D212) (refs 3 , 4 ), and (ii) carboxylates in the loops, the potential candidates of sodium ion-binding site ( Fig. 5a ). All mutants were expressed enough to apply pump measurements, though E160Q was not stable in detergent ( Supplementary Fig. S13 ). Supplementary Figure S14 shows that large spectral red shift was observed only for D116N and D116A, but not D116E, implying that D116 in the NDQ motif is the RSB counterion. It should be noted that almost no colour changes were observed for the D251 mutants, though D212 in BR functions as the RSB counterion [35] . We also determined the molar extinction coefficients of wild type (WT) and mutants, which ranges 30,000–50,000 ( Supplementary Fig. S15 ), and these values were used for quantifying the pump activity measurements ( Supplementary Figs S16 and S17 ). 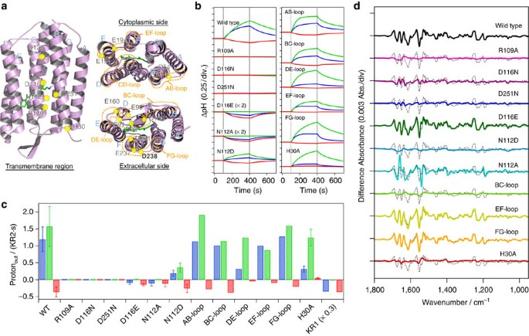Figure 5: Mutational analysis to of KR2. (a) Positions of mutated amino-acid residues (yellow spheres) based on the crystal structure of BR55. We introduced D/N and E/Q mutations into carboxylates at each loop. (b) pH changes caused by light-driven ion pump ofE. colicells suspensions expressing KR2 mutants. The solution contains 100 mM NaCl (blue lines), after addition of CCCP (green lines) and 100 mM KCl (red lines). Light was turned on and off att=100 s and 400 s, respectively. (c) Quantitatively normalized pump activities of each mutant estimated from the initial slope of light-induced pH changes. Positive and negative signals represent outward sodium pump with subsequent secondary proton uptake and outward proton pump activities, respectively. (d) ATF-FTIR difference spectra of KR2 mutants upon the exchange of 50 mM NaCl/KCl. Figure 5: Mutational analysis to of KR2. ( a ) Positions of mutated amino-acid residues (yellow spheres) based on the crystal structure of BR [55] . We introduced D/N and E/Q mutations into carboxylates at each loop. ( b ) pH changes caused by light-driven ion pump of E. coli cells suspensions expressing KR2 mutants. The solution contains 100 mM NaCl (blue lines), after addition of CCCP (green lines) and 100 mM KCl (red lines). Light was turned on and off at t =100 s and 400 s, respectively. ( c ) Quantitatively normalized pump activities of each mutant estimated from the initial slope of light-induced pH changes. Positive and negative signals represent outward sodium pump with subsequent secondary proton uptake and outward proton pump activities, respectively. ( d ) ATF-FTIR difference spectra of KR2 mutants upon the exchange of 50 mM NaCl/KCl. Full size image Both sodium ion and proton-pumping activities are completely lost for R109A, D116N and D251N ( Fig. 5b ). ATR-FTIR shows that sodium ion binding is lost for R109A ( Fig. 5d ), indicating that R109 is prerequisite for sodium ion–proton pumps and sodium ion binding. Figure 5d shows that sodium ion binding is weak but still substantial for D116N and D251N, suggesting that D116 and D251 are key residues for pump, but sodium ion binding is possible for these mutants. The photocycle of D116N, the RSB counterion mutant, exhibits only a red-shifted intermediate ( Supplementary Fig. S18 ), which is similar to the case of the WT at pH 3.6 ( Supplementary Fig. S19 ). Thus, D116 is important for the formation of the blue-shifted intermediate ( Fig. 4 ), which is prerequisite for the sodium ion pump. In other words, D116 is suggested to function as the proton acceptor from RSB, by which neutralized RSB region allows uptake of a sodium ion from the cytoplasmic side. We found that D116E and N112A mutants abolish sodium ion pump activity, but they pump proton even in NaCl. ATR-FTIR shows that the structure of the sodium ion-binding site of D116E is identical to that of WT, while largely modified for N112A. In case of D116E, sodium ion binding is normal, but sodium ion pump function is lost, suggesting that the pore size for sodium ion transport may become too narrow by the D-to-E mutation. This further suggests that D116 constitutes the selectivity filter of ions. The pump property of N112D was similar to that of WT ( Fig. 5b ), but ATR-FTIR shows no sodium ion binding ( Fig. 5d ). This is a surprising result, because normal sodium ion pump takes place even without sodium ion binding. This suggests that sodium ion binding is not the requirement of the sodium ion pump. As 11 carboxylates near the surface are the potential candidates for the sodium ion-binding site, we introduced D/N and E/Q mutations for each loop (AB, BC, DE, EF and FG loops). The loop mutants all showed normal hybrid sodium ion–proton pump ( Fig. 5b ), but interestingly, ATR-FTIR shows no sodium ion binding to the BC-loop mutant (E90Q/E91Q/D98N/D102N) ( Fig. 5d ). Loss of sodium ion binding ( Fig. 5d ) suggests that R109, N112 and carboxylates in BC-loop constitute the sodium ion-binding site ( Fig. 6 ). 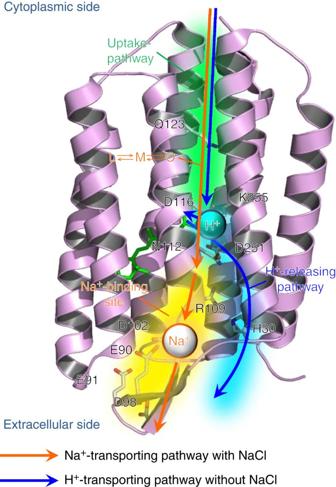Figure 6: Model for sodium ion and proton pumpings by KR2. KR2 is considered to pump a sodium ion in marine environment, and proton is pumped in the absence of sodium ion or lithium ion. R109 and carboxylates in BC-loop at residues E90, E91, D98 and D102 constitute binding site of the sodium ion, while H30 is important for proton pump. Figure 6: Model for sodium ion and proton pumpings by KR2. KR2 is considered to pump a sodium ion in marine environment, and proton is pumped in the absence of sodium ion or lithium ion. R109 and carboxylates in BC-loop at residues E90, E91, D98 and D102 constitute binding site of the sodium ion, while H30 is important for proton pump. Full size image While D116E and N112A are converted from the hybrid sodium ion–proton pump to uni-functional proton pump, we found that the H30A mutant becomes uni-functional sodium ion pump ( Fig. 5b ). This indicates that H30 in A-helix is required for proton pumping, which is presumably located in the hydrogen-bonding network. Functionally important residues of KR2 such as R109, N112, D116 and D251 are also important for other microbial rhodopsins (R82, D85, T89 and D212 in BR) [26] , [36] , [37] , [38] , whereas H30 is a unique residue in KR2. Interestingly, H30A pumps the sodium ion, but its binding signal is unclear ( Fig. 5d ). Thus, H30A, N112D and BC-loop mutant have no sodium ion-binding site, but they can pump sodium ion. This again suggests that sodium ion binding is not required for sodium ion pump. K. eikastus KR2 is a hybrid outward sodium ion–proton pump in the marine flavobacteria. Nature creates and utilizes a light-driven sodium ion pump in the ocean in a manner similar to other membrane transporters. Little colour change between the presence and absence of sodium ion ( Fig. 3a and Supplementary Fig. S7 ) shows that the binding site is distant from the retinal chromophore. Mutation study indeed suggested that the sodium ion-binding site is comprised of R109, N112 and carboxylates in BC-loop ( Fig. 5 ). We infer direct sodium ion binding to carboxylates in BC-loop, which is stabilized by hydrogen-bonding network extended to R109 and N112 ( Fig. 6 ). It should be noted that the sodium ion-binding site is not required for sodium ion pump, suggesting that the sodium ion-binding site is transiently formed in the cytoplasmic domain. Transient helix opening probably occurs during the photocycle in a manner similar to other microbial rhodopsins [39] , [40] , [41] , [42] , and we expect such helical movement produces transient binding site for sodium ion uptake. Transient absorption study monitored the formation of common photointermediates (K, L, M and O states; Fig. 4 ) in microbial rhodopsins [3] , [4] , among which the sodium ion uptake from the cytoplasmic side accompanies the O formation ( Supplementary Fig. S11 ). Deprotonation of RSB (M formation) is presumably prerequisite for the sodium ion uptake, because D116N exhibits neither M formation nor sodium ion pump ( Supplementary Fig. S18 ). Therefore, the proton transfer from RSB to D116 lowers the potential barrier for the sodium ion uptake in the cytoplasmic domain. Regarding the O intermediate, charge balance near RSB is important. The O intermediate has protonated D85 for BR [43] and chloride unbound for HR [23] , [24] , where the total electric charge is +1 compared with the initial state. Thus, sodium ion may be located near RSB in the O intermediate of NaR, where a positive charge near the protonated RSB causes a spectral red shift. ChR, a light-gated cation channel, also transports sodium ion in a passive manner [23] , [24] , whereas NaR, a sodium ion pump, undergoes an active transport. Therefore, the mechanistic comparison is intriguing between sodium ion channel and pump. Recent X-ray structure of ChR suggests the sodium ion transport pathway, which does not include the RSB region [8] . In contrast, the RSB region is likely to constitute the sodium ion transport pathway in NaR ( Fig. 6 ). This sounds reasonable, because ChR transports multiple cations upon channel opening, but sodium ion pump needs a specific machinery to inhibit backward flow. In KR2, D116 and N112 probably determine the pore size of transported cations. KR2 pumps proton when presented with KCl or salts of larger cations, but proton pump efficiency (16 proton KR2 −1 min −1 ) is much lower than other prototypical proton pumps (100–200 proton molecule −1 min −1 ). As KR2 functions as a sodium ion pump under physiological marine environment, this molecule has optimized the sodium ion-pumping machinery. In other words, this may suggest that proton pump is an evolutional origin of sodium ion pump. Although similar photointermediates appear, proton-pumping photocycle is slower than that of Na + pump ( Fig. 4 ). Slow photocycle is mainly because Q123 in KR2 (D96 in BR) cannot be a proton donor to RSB. Q123D and Q123E exhibit improved proton pumps ( Supplementary Figs S16 and 17 ), whereas the improvement is not so significant. Interestingly, proton pump activity is lost in H30A ( Fig. 5 ), which also abolishes sodium ion binding, but sodium ion pump is preserved. Thus, sodium ion and proton transport pathways are mostly common in KR2, and more detailed mechanism will be studied in future. KR2 is a hybrid outward sodium ion–proton pump in the marine flavobacteria. NaR probably contributes to generate membrane potential using light energy and also has a key role to maintain intracellular low sodium ion concentration. In this regard, excretion of the lithium ion by light is potentially important, because the lithium ion is poisonous to cells [44] . In addition, controlled intracellular sodium ion concentration by KR2 may be correlated to the growth of the marine flavobacteria, which is suggested by its expression at the early phase of the growth ( Fig. 1a ). In contrast, a light-driven proton pump KR1 grows slowly, suggesting different functional roles other than generation of membrane potential. After submission of this paper, one paper was reported in which the presence of a light-driven sodium ion pump was proposed based on an enhanced expression of a marine bacterium at high salt concentration [45] . The present results are fully consistent with their proposal, and a light-driven sodium ion pump is now experimentally proven. Finding of the light-driven sodium ion pump will lead to better understanding of physiology of marine microbes [46] , and molecular mechanism of light-driven pumps. Finally, the hybrid sodium ion–proton pump will contribute to the development of new optogenetic tools. Optogenetics revolutionized neuroscience research using light to control animal behaviour [6] , [7] , [8] , [9] , and light-driven proton and chloride pumps have been so far used as neural silencers [10] , [11] . The hybrid sodium ion–proton pump will be a promising neural silencer, whose function could be flexibly controlled by the environment. Bacterial strains and sequencing of KR1 and KR2 from K. eikastus NBRC100814 T K. eikastus NBRC 100814 T was purchased from NITE Biological Resource Center, National Institute of Technology and Evaluation in Japan. Full-length sequence of KR1 and KR2 was determined with the primer sets of KrokinoR1 F/R and KrokinoR2 F/R. These were designed by reference to whole genome data of Krokinobacter sp. 4H-3-7-5 (NC_015496). The sequences were deposited in DDBJ/EMBL/GenBank (accession nos. KR1: AB738959 and KR2: AB738960 ). Phylogenetic analysis We constructed phylogenies with MEGA5 software [47] . The protein sequences were aligned using MUSCLE [48] . The evolutionary distances were calculated with the JTT matrix-based method [49] . We clustered data by Neighbour-Joining [50] , with bootstrap values based on 1,000 replications [51] . Sequence data of the other rhodopsins were from the GenBank database. Cloning and expression of KR1 and KR2 from K. eikastus NBRC100814 T Routine DNA manipulations were carried out according to standard procedures. The genes for KR1 and KR2 were amplified using PCR from the genome of K. eikastus . The forward primers for KR1 and KR2, 5′-AAGGAGATATA CATATG AAATTTTTATTACTATTAC-3′ and 5′-AAGGAGATATA CATATG ACACAAGAACTAGGGAATGCC-3′ and the reverse primers for KR1 and KR2, 5′-GGTGGTGGTG CTCGAG AACAACATCAACTTCATTC-3′ and 5′-GGTGGTGGTG CTCGAG GCTATTTGCTTCAACCAAC-3′ were designed (underlining indicates the restriction site for Nde I and Xho I, respectively). These fragments were inserted to Nde I and Xho I sites of pET21a vector (Novagen). Consequently, the plasmid encodes hexahistidines at the C terminus. A point mutation was introduced into the KR2 gene by PCR mutagenesis (Stratagene). The constructed plasmids were analyzed using an automated sequencer to confirm the expected nucleotide sequence. Measurement of light-driven pump activity of K . eikastus K. eikastus was grown aerobically in Marine Broth 2216. Overnight cultures were diluted 1:50 and cultures were grown in shaker flasks at 20 °C for each time at 125 r.p.m. Growths were monitored by measuring the optical density of culture at 660 nm (OD 660 ) with miniphoto518R (TAITEC, Japan). Light-driven pump activity was measured by monitoring pH changes in the suspensions [17] . The cells were collected by centrifugation (10,000 g , 10 min), washed once in 100 mM NaCl, resuspended in 100 mM NaCl and adjusted to OD 660 =8.5. Six millilitres of cell suspension were first placed in darkness and then illuminated using outputs of a 1 kW tungsten–halogen projector lamp (Master HILUX-HR, Rikagaku, Japan) through a glass filter (Y-52, AGC Techno Glass, Japan) for 5 min at wavelengths >500 nm. pH changes during incubation were monitored with a pH meter (F-55, Horiba, Japan). Measurements were repeated under the same conditions after addition of CCCP and further addition of TPP + . Measurement of light-driven pump activity heterologously expressed rhodopsins in E. coli E. coli expressing rhodopsins was prepared in manner previously described [52] , [53] . The cells were collected by centrifugation (4,800 g , 3 min), washed three times and resuspended in the solvent for measurement. Seven point five millilitres of cell suspension was placed in darkness and then illuminated using outputs of a 1-kW tungsten–halogen projector lamp (Master HILUX-HR, Rikagaku, Japan) or a 100-W Xe arc lamp (LM103, ASAHI spectra, Japan) through a glass filter (Y-52, AGC Techno Glass, Japan) for 5 min at wavelengths >500 nm. The light-induced pH changes were measured under 100 mM salt concentrations as described for the K. eikastus cell suspensions. Protein expression in E. coli and purification KR1 and KR2 having six histidines at the C terminus were expressed in E. coli C41(DE3) strain. The protein was purified via Co-affinity column (TALON, Qiagen) chromatography in manner previously described [52] , [53] and solubilized in 0.1% n -dodecyl-β- D -maltoside (DDM). ATR-FTIR measurement For ATR-FTIR measurement, KR2 was reconstituted into 1,2-dioleoyl-sn-glycero-3-phosphocholine (DOPC; molar ratio was KR2:DOPC=1:20). The sample was placed on the surface of a diamond ATR crystal (nine internal total reflections). After being dried in a gentle stream of N 2 , the sample was rehydrated with first solvent containing 50 mM NaCl, 5 mM Tris–HCl (pH 8.0) at a flow rate of 0.5 ml min −1 . ATR-FTIR spectra was recorded at 2 cm −1 resolution with an FTIR spectrometer (Agilent, CA, USA) equipped with a liquid nitrogen-cooled MCT detector [31] . After exchanging to second solvent and recording FTIR spectrum, the difference FTIR spectrum was calculated by the subtraction between the data obtained for first and second solvents. Flash photolysis The transient absorption spectra of rhodopsins were monitored by flash photolysis measurements using a multichannel detector (Hamamatsu Photonics, Japan) [54] . The purified sample was resuspended in buffer containing 50 mM Tris–HCl (pH 8.0), 100 mM salt (NaCl, KCl or LiCl) and 0.1% DDM. The sample solution was placed in a quartz cuvette and it was illuminated with a beam of second harmonics of a nanosecond pulsed Nd 3+ -YAG laser ( λ =532 nm, INDI40, Spectra-Physics). The laser power was 300 μJ per pulse, and repetition rate was sufficiently slower than the rate of photocycle of rhodopsin to avoid photo-excitation of transient intermediates. The intensities of the transmitted probe light from a Xe arc lamp (L8004, Hamamatsu Photonics, Japan) were measured before and after laser excitation, and transient absorption spectra were obtained by calculating the ratio between them. Thirty to fifty identical spectra were averaged. To obtain the time-evolution of absorption at specific wavelengths, absorption change after laser excitation was probed by monochromated light from the output of a Xe arc lamp (L9289-01, Hamamatsu Photonics, Japan), and the change of the intensity of probe light passed through the sample was monitored by a photomultiplier tube (R10699, Hamamatsu Photonics, Japan). The signal from the photomultiplier tube was averaged and stored by a digital-storage-oscilloscope (DPO7104, Tektronix, Japan). Quantification of rhodopsin expressed in E. coli E. coli cell expressing rhodopsin was centrifuged and suspended in the solvent containing 100 mM NaCl, 50 mM Tris–HCl (pH 8.0) to final volume of 3 ml. Then, 200 μl of 1 mM lysozyme and 200 μl of 20 mM DNase were added. E.coli cell was disrupted by ultrasonication, and rhodopsin was solubilized in 2.0% DDM. The cell debris was removed by ultracentrifuge after solubilization. Absorption change representing the bleaching of rhodopsin by the hydroxylamine were measured by ultraviolet–visible spectrometer for 0.5–1.5 h after the addition of hydroxylamine to final concentration of 500 mM under the illumination by a output from a 1-kW tungsten–halogen projector lamp (Master HILUX-HR, Rikagaku, Japan) through a glass filter (Y-52, AGC Techno Glass, Japan) at wavelengths >500 nm. Molecular extinction coefficient of rhodopsin ( ε ) was calculated by the ratio between absorbance of rhodopsin and retinal oxime ( ε =33,900 M −1 cm −1 ) and the amount of rhodopsin expressed in E. coli cell was determined by absorbance of bleached rhodopsin and the ε . How to cite this article: Inoue, K. et al . A light-driven sodium ion pump in marine bacteria. Nat. Commun. 4:1678 doi: 10.1038/ncomms2689 (2013).